Single-cell transcriptomics uncovers a non-autonomousTbx1-dependent genetic program controlling cardiac neural crest cell development Disruption of cardiac neural crest cells (CNCCs) results in congenital heart disease, yet we do not understand the cell fate dynamics as these cells differentiate to vascular smooth muscle cells. Here we performed single-cell RNA-sequencing of NCCs from the pharyngeal apparatus with the heart in control mouse embryos and when Tbx1 , the gene for 22q11.2 deletion syndrome, is inactivated. We uncover three dynamic transitions of pharyngeal NCCs expressing Tbx2 and Tbx3 through differentiated CNCCs expressing cardiac transcription factors with smooth muscle genes. These transitions are altered non-autonomously by loss of Tbx1 . Further, inactivation of Tbx2 and Tbx3 in early CNCCs results in aortic arch branching defects due to failed smooth muscle differentiation. Loss of Tbx1 interrupts mesoderm to CNCC cell-cell communication with upregulation and premature activation of BMP signaling and reduced MAPK signaling, as well as alteration of other signaling, and failed dynamic transitions of CNCCs leading to disruption of aortic arch artery formation and cardiac outflow tract septation. Neural crest cells (NCCs) are multipotent cells that migrate in three ordered streams from the rhombomeres in the neural tube to the pharyngeal apparatus, where they differentiate into many cell types [1] . The pharyngeal apparatus is a dynamic embryonic structure consisting of individual pharyngeal arches (PA), forming in a rostral to caudal manner from mouse embryonic day (E) 8 to E10.5. A subset of pharyngeal NCCs migrate through the caudal pharyngeal arches, PA3-6, and surround the pharyngeal arch arteries (PAAs), while others continue to migrate to the cardiac outflow tract (OFT), both differentiating to vascular smooth muscle cells [2] . The PAAs form in a similar, rostral to the caudal manner and are linked continuously with the cardiac OFT. The PAAs become remodeled to form the aortic arch and vascular branches that include the subclavian arteries. The fourth PAAs are particularly important in that the left fourth PAA is critical to form the aortic arch with the left subclavian artery and the right fourth PAA forms the branch to the right subclavian artery. Differentiation of CNCCs into smooth muscle cells of the PAAs is important for the remodeling of the PAA [2] . The OFT elongates by the addition of second heart field mesoderm cells and this is required for looping and septation of the OFT. It has been shown that CNCCs are required for the addition of second heart field mesoderm cells to expand the length of the OFT [3] . In addition, CNCCs are required for OFT septation by invading and allowing the endocardial cushions of the OFT to come into direct cell-cell contact, fuse, and form the aorticopulmonary septum [2] , [4] , [5] . Complete ablation of NCCs from PA3-6 results in interruption of the aortic arch and arterial branching defects, as well as persistent truncus arteriosus of the OFT [6] . These NCCs in PA3-6, are referred to as cardiac NCCs (CNCCs) based upon their position and known function in heart development as well as their differentiation to vascular smooth muscle. Understanding CNCC development is critical to determine the pathogenesis of human congenital heart defects such as those observed in 22q11.2 deletion syndrome (22q11.2DS) patients [7] , [8] . TBX1 , encoding a T-box transcription factor, is the major gene for congenital heart disease in 22q11.2DS. Although 22q11.2DS is largely considered to be a neurocristopathy, Tbx1 is not significantly expressed in CNCCs [9] , but it is strongly expressed in adjacent cells in the pharyngeal apparatus, including the mesoderm. Global inactivation of Tbx1 or conditional inactivation in the mesoderm using Mesp1 Cre [10] in the mouse results in neonatal lethality with a persistent truncus arteriosus [11] , [12] , [13] , in part due to failed CNCC development [9] . Therefore, one of the main functions of Tbx1 in the pharyngeal mesoderm is to signal to CNCCs to promote their development. In order to understand how CNCCs are affected non-autonomously in Tbx1 mutant embryos, it is essential to define their transcriptional signatures and cardiac fate acquisition in the normal situation between E8.5 and E10.5, when Tbx1 is expressed in the pharyngeal apparatus and when inactivated, on a single-cell level. Previously, single-cell RNA-sequencing (scRNA-seq) of NCCs from early stages in the chick embryo identified expression of Tgif1 , Ets1 , and Sox8 being important for early CNCC identity and fate decisions [14] . However, these were early migrating mesenchymal NCCs that also have the potential to contribute to the craniofacial skeleton and other cell types. Another seminal scRNA-seq study demonstrated that NCC fate choices are made by a series of sequential binary decisions in mouse embryos at E8.5-10.5 [15] but did not focus on detailed steps of cardiac fate acquisition or investigate Tbx1 function [15] . In another recent study using mouse scRNA-seq data, Chen and colleagues focus on CNCC differentiation from E10.5 to P (postnatal day) 7, once Wnt1-Cre derived NCCs have migrated to their final destinies in the heart [16] . However, this study did not include an analysis of the cardiac progenitor cells in the pharyngeal arches. To uncover genetic signatures and dynamic transitions of CNCCs in the normal situation and when Tbx1 is inactivated, we performed scRNA-seq of NCCs from control and Tbx1 null mutant mouse embryos. We found that smooth muscle cell fate acquisition is in part dependent on two other T-box genes, Tbx2 and Tbx3 . When Tbx1 is inactivated, we found reduced cell deployment (reduced presence of cells) along with the failure of dynamic progression of CNCC maturation. This is due to the disruption of cell-cell communication from mesodermal cells, resulting in the downregulation of MAPK signaling and upregulation and premature activation of the BMP pathway, as well as affecting other ligand–receptor interactions. Single-cell transcriptional profiling of NCCs in the pharyngeal apparatus We performed scRNA-seq of the Wnt1-Cre;ROSA-EGFP genetic lineage [17] , [18] in the mouse pharyngeal apparatus at E8.5, E9.5 and E10.5 (Fig. 1a–f ). These stages correspond to developmental time points when Tbx1 is highly expressed in cell types adjacent to NCCs. At E8.5, the anterior half of the embryo was dissected and used for the scRNA-seq experiment because the embryo was too small to microdissect the pharyngeal apparatus with heart (Fig. 1a ). At E9.5, the pharyngeal apparatus with heart was microdissected with the neural tube at the level of the pharyngeal apparatus, excluding the head and caudal half of the embryo in order to enrich for NCCs relevant to the PAAs and heart (Fig. 1b ). At E10.5, the first arch, PA1 is large in size in proportion to the rest of the pharyngeal apparatus and contains NCCs that contribute to the craniofacial skeleton. We excluded PA1 in order to enrich for NCCs relevant to cardiac development. At E10.5, arches two to six and the heart were included in the dissection (Fig. 1c ). 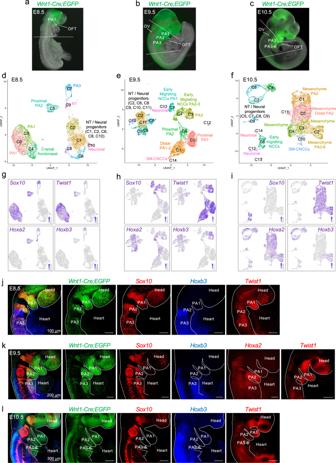Fig. 1: Single-cell RNA-seq of NCCs from mouse embryos at E8.5-E10.5 reveals transcriptional heterogeneity within the pharyngeal region. a–cWnt1-Cre;ROSA-EGFPgenetic lineage tracing shows the distribution of NCCs within the pharyngeal region and outflow tract of E8.5 (a), E9.5 (b), and E10.5 (c) embryos. The region rostral to the white dotted line of the embryo at E8.5 (a) and the pharyngeal region between the dotted lines in embryos at E9.5 and E10.5, including the heart were microdissected and EGFP-positive NCCs were used for scRNA-seq.d–fSeurat UMAP (Uniform Manifold Approximation and Projection) plots with cluster annotations of scRNA-seq data of NCCs at E8.5 (d), E9.5 (e), and E10.5 (f).g–iExpression of genes at E8.5 (g), E9.5 (h), and E10.5 (i) with highest expression in blue and lowest expression in gray.j–lWholemount RNAscope in situ hybridization ofWnt1-Cre;ROSA-EGFPembryos (n= 3) at E8.5 (j), E9.5 (k), and E10.5 (l) with probes forSox10,Hoxb3, andEgfp, together and separated (colors are indicated above embryos).Twist1expression was analyzed at E8.5, E9.5, and E10.5 andHoxa2was examined at E9.5 as indicated. PA pharyngeal arch, OFT outflow tract, OV otic vesicle, SM-CNCCs smooth muscle CNCCs. Scale bar: 100 μm inj, 200 μm ink, and 300 μm inl. EGFP-positive NCCs were purified by FACS and the Chromium 10X platform was used to perform scRNA-seq and data from 36,721 NCCs of control embryos were obtained (Supplementary Table 1 ). Unsupervised clustering was performed using Seurat software [19] and individual clusters were identified (Fig. 1d–f and Supplementary Figs. 1 – 3 ). Fig. 1: Single-cell RNA-seq of NCCs from mouse embryos at E8.5-E10.5 reveals transcriptional heterogeneity within the pharyngeal region. a – c Wnt1-Cre;ROSA-EGFP genetic lineage tracing shows the distribution of NCCs within the pharyngeal region and outflow tract of E8.5 ( a ), E9.5 ( b ), and E10.5 ( c ) embryos. The region rostral to the white dotted line of the embryo at E8.5 ( a ) and the pharyngeal region between the dotted lines in embryos at E9.5 and E10.5, including the heart were microdissected and EGFP-positive NCCs were used for scRNA-seq. d – f Seurat UMAP (Uniform Manifold Approximation and Projection) plots with cluster annotations of scRNA-seq data of NCCs at E8.5 ( d ), E9.5 ( e ), and E10.5 ( f ). g – i Expression of genes at E8.5 ( g ), E9.5 ( h ), and E10.5 ( i ) with highest expression in blue and lowest expression in gray. j – l Wholemount RNAscope in situ hybridization of Wnt1-Cre;ROSA-EGFP embryos ( n = 3) at E8.5 ( j ), E9.5 ( k ), and E10.5 ( l ) with probes for Sox10 , Hoxb3 , and Egfp , together and separated (colors are indicated above embryos). Twist1 expression was analyzed at E8.5, E9.5, and E10.5 and Hoxa2 was examined at E9.5 as indicated. PA pharyngeal arch, OFT outflow tract, OV otic vesicle, SM-CNCCs smooth muscle CNCCs. Scale bar: 100 μm in j , 200 μm in k , and 300 μm in l . Full size image Expression of Sox10 and Foxd3 , as well as expression of Twist1, Prrx1 , and Prrx2 were used to identify early migratory and mesenchymal NCCs, respectively [20] , [21] . We used Hox and Dlx (Homeodomain) genes to provide spatial anterior-posterior and proximal-distal context to different arches (PA2-6 [22] ). At E8.5, Sox10 and Twist1 show overlap in expression, while at E9.5, the expression became complementary, with a relative reduction of Sox10 + NCCs and increased Twist1 + NCCs in the expanded populations of mesenchymal NCCs (Fig. 1g, h ). At E8.5 and E9.5, Hoxa2 was expressed in PA2 and caudal arches, while Hoxb3 was expressed only in PA3 and more caudal arches containing NCCs that will invade the OFT and surround the PAAs (Fig. 1d, e, g, h ). Using the Hox genes as a guide, at E9.5, early migrating Sox10 + NCCs of PA2 and PA3 were clustered together (cluster C4), suggesting that they have a similar transcriptional profile. At E10.5, the relative proportion of Twist1 -expressing mesenchymal cells increased with respect to the reduction of Sox10- expressing cells (Fig. 1f, i ). Further, at E10.5, Hoxa2 was expressed within the mesenchymal cell populations from PA2-6, and Hoxb3 was expressed in NCCs of PA3-6 (Fig. 1f, i ). Additional marker genes are shown in Supplementary Fig. 1 (E8.5), Supplementary Fig. 2 (E9.5), and Supplementary Fig. 3 (E10.5) and listed in Supplementary Data 1 (E8.5), 2 (E9.5), and 3 (E10.5). Spatial localization was confirmed for expression of S ox10 , Hoxa2 , Hoxb3 , and Twist1 by wholemount RNAscope in situ hybridization (Fig. 1j–l ). In addition, to anterior-posterior spatial localization of the cells, we identified their proximal-distal location in the PAs with Dlx2 , Dlx5 , and Dlx6 (Supplementary Fig. 4 ). NCCs of the neural tube were identified based on the expression of Zic1 and Zic2 genes and additional neural gene markers (Supplementary Figs. 1 – 3 and Supplementary Data 1 – 3 ). Identification of cardiac NCC gene signatures Differentiated NCCs of the OFT and PAAs express smooth muscle genes such as smooth muscle actin, Acta2 [23] , [24] . Acta2 is a representative marker gene of progenitor smooth muscle cells, but it is not exclusive to smooth muscle cell types. Early markers of smooth muscle cells in addition to Acta2 are Tagln , Myl9 , Myh9 , Rgs5 , and Cnn1 [25] , [26] , [27] . We used Tagln (Transgelin), Cnn1 (Calponin), and Rgs5 (Regulator of G Protein Signaling 5) as markers (Figs. 2 , 3 ). CNN1 is a basic smooth muscle protein [28] , RGS5 is expressed in vascular smooth muscle and pericytes [29] and TAGLN is ubiquitously expressed in vascular smooth muscle cells and is an early marker of smooth muscle differentiation [30] . This cell population also expresses additional markers of smooth muscle progenitors (Supplementary Data 3 ). By combining results from Wnt1-Cre;GFP lineage tracing experiments, immunofluorescence, and RNAscope experiments of the early smooth muscle genes (cluster C14, Fig. 2a ; C10, Fig. 3a ; and Supplementary Figs. 2, 3 ), we refer to these cells as SM-CNCCs (smooth muscle expressing CNCCs). Furthermore, we performed co-immunostaining at E10.5 for Wnt1-Cre;GFP , ACTA2, and MF20 (myosin heavy chain antibody) to discriminate cardiac skeletal muscle cells, that also express ACTA2, from adjacent SM-CNCCs in the OFT. Supplementary Fig. 5 shows that MF20 is detected, as expected, in cardiac skeletal muscle cells but not in SM-CNCCs of the OFT. Fig. 2: Transcriptional dynamics of cardiac NCCs at E9.5. a UMAP plots of scRNA-seq data with genes that mark CNCCs identified by expression of Acta2 , Isl1 , Gata3 , Hand2 , Msx2 , Tbx2 , and Tbx3 with respect to Hoxb3 (PA3) and Dlx5 (distal PA1, 2, 3) expression (red arrows). Blue arrows show the expression of Gata3 , Hand2 , Msx2 , Tbx2 , and Tbx3 in the distal part of PA3. b , c Immunostaining on traverse sections through Wnt1-Cre;ROSA-EGFP embryos showing Cre -activated EGFP (green), ACTA2, TAGLN, and ISL1 protein expression. Nuclei (blue) are labeled with DAPI. White arrowheads indicate CNCCs expressing ACTA2 and ISL1 ( n = 3) ( b ) and CNCCs expressing TAGLN ( n = 3) ( c ) in the OFT. d – f RNAscope analysis of Wnt1-Cre;ROSA-EGFP embryos for Egfp , Gata3 ( d ) ( n = 3), Isl1 ( e ) ( n = 3), and Msx2 ( f ) ( n = 4) expression. Nuclei (blue) are labeled with DAPI. Arrowheads indicate the expression of Gata3 , Isl1 , and Msx2 in CNCCs within the OFT. g Wholemount RNAscope analysis of Wnt1-Cre;ROSA-EGFP embryos at 20 and 24 somites where the position of the OFT is indicated (white arrowhead). h PHATE (potential of heat-diffusion for affinity-based transition embedding) map of NCCs in clusters C1, C3, C4, C5, and C14 using Louvain clustering. i PHATE map colored by cell fate probabilities, showing how each cell is likely to transition to SM-CNCCs as defined by CellRank software (yellow represents high cell fate probabilities). j Heatmap from CellRank showing the expression of marker genes whose expression correlates with cardiac fate probabilities as latent time, with cells order by fate probabilities as latent time (see Supplementary Data 4 for a full list of genes), Asterisk (*) indicates newly identified genes connected to CNCCs. k PHATE maps with an expression of marker genes of CNCCs at different states of differentiation towards smooth muscle Acta2 expressing cells. NT neural tube, end endoderm, OFT outflow tract, PA pharyngeal. Scale bars: 100 μm. Full size image Fig. 3: Transcriptional dynamics of cardiac NCCs at E10.5. a Seurat UMAP plots of scRNA-seq data from NCC populations with the expression of marker genes. b Immunostaining on traverse sections of Wnt1-Cre;ROSA-EGFP embryos ( n = 3) showing GFP, ISL1, and ACTA2 expression. Nuclei stained with DAPI are in blue. ISL1 is expressed in smooth muscle cells of the OFT cushions (arrowheads). c – e RNAscope in situ hybridization sections of Wnt1-Cre;ROSA-EGFP embryos for Egfp , Isl1 and Gata 3 ( c ) ( n = 5), Egfp , Cnn1 ( d ) ( n = 3), Egfp and Rgs5 ( e ) ( n = 3) expression. Nuclei stained with DAPI are in blue. Isl1 and Gata3 are expressed in NCCs within the OFT (white arrowheads in c ) and at the level of the dorsal aortic sac wall and aortic sac protrusion (blue arrowheads in c ). Gata3 but not Isl1 is expressed in the more proximal part of OFT (red arrowheads in c ). Cnn1 and Rgs5 are expressed in smooth muscle cells of the OFT (white arrowheads in d and e ). f Immunostaining on sections of Wnt1-Cre;ROSA-EGFP embryos ( n = 3) showing GFP, TBX2, and TAGLN expression. Expression of TAGLN is in smooth muscle cells of the OFT (blue arrowheads) and PAAs expressing TBX2 (white arrowheads). g – i RNAscope in situ hybridization on traverse sections of Wnt1-Cre;ROSA-EGFP embryos for Egfp , Tbx2 ( n = 5) and Gata3 ( n = 4) ( g ), Egfp and Tbx2 ( h ) ( n = 5), and Egfp and Tbx3 ( i ) ( n = 5) expression. Nuclei stained with DAPI are in blue. Tbx2 and Gata3 expression overlaps in the dorsal wall of the OFT (white arrowheads in g ). Tbx2 and Tbx3 are expressed in the mesenchyme dorsal to the aorta surrounding the PAAs at the level of the PA3-6 (white arrowheads in h and i ). j Schematic representation of a transverse section at the level of the OFT summarizing Tbx2 , Tbx3 , Isl1 , Gata3 , Acta2 , and Tagln expression in CNCCs at E10.5. NT neural tube, end endoderm, PAA pharyngeal arch artery. Scale bars: 100 μm. Full size image To further delineate molecular signatures of CNCCs, we evaluated genes that were co-expressed in the SM-CNCCs (cluster C14, Fig. 2a ; cluster C10, Fig. 3a ). We identified known transcription factor genes involved in cardiac development, but not all of these are known to have a function in CNCCs development, including Tbx2, Tbx3, Msx2, Isl1 , Gata3 , and Hand2 , at E9.5 and E10.5 (Figs. 2a , 3a ). These genes were not only expressed in SM-CNCCs of the OFT but also in other cell clusters, such as NCCs in the distal PA1-3 expressing Dlx5 at E9.5 (C1, C3; Fig. 2a ) and in PA3-6 at E10.5 (C2, C3, C4; Fig. 3a ). At E9.5, we validated the expression of ACTA2 and TAGLN in SM-CNCCs in the distal part of the OFT (Fig. 2b, c ) and co-expression of ISL1 in SM-CNCCs of which some expressed ACTA2 (Fig. 2b ). Further, RNAscope in situ analysis confirmed the expression of Gata3 , Isl1 , and Msx2 in CNCCs within the OFT at E9.5 (Fig. 2d–f ). At E10.5, Isl1 and Gata3 were expressed in CNCCs in the OFT and some also expressed ACTA2, Cnn1 , Rgs5 , and TAGLN (Fig. 3a–f ) within the cardiac cushions of the distal OFT and in the mesenchyme of the dorsal aortic sac wall and aortic sac protrusion. Gata3 was expressed in a larger domain of the OFT than Isl1 (Fig. 3c ). When taken together, at this time point, CNCCs of the OFT derived from the Wnt1-Cre;GFP genetic lineage and expressing Acta2 , Tagln , Cnn1 , Rgs5 , Isl1 , and Gata3 are smooth muscle progenitors. Tbx2 and Tbx3 were widely expressed in pharyngeal NCCs at E9.5 (Fig. 2a ), but their expression was restricted to cell clusters comprising PA3-6 at E10.5 (Fig. 3a ). Tbx2 and Tbx3 were expressed immediately lateral and dorsal to Isl1 and Gata3 expressing CNCCs in embryos at E10.5 as determined by RNAscope analysis (Fig. 3g–i ). A Tbx2 and Gata3 co-expression domain was present between Tbx2 and Gata3 expressing CNCCs (Fig. 3g ). Together, this suggests that CNCCs downregulate Tbx2 and Tbx3 expression and activate Isl1 and Gata3 expression when entering the OFT. In addition, Tbx2 and Tbx3 , but not Isl1 and Gata3 , were expressed in NCCs surrounding the PAAs that are differentiating to smooth muscle, expressing ACTA2 and TAGLN at E10.5 (Fig. 3f, h, i ). Both ISL1 and TBX2 proteins were expressed in smooth muscle cells of the OFT and PAAs, respectively (ACTA2 or TAGLN; Fig. 3b, f ). Expression of Tbx2 , Tbx3 , Isl1 , Gata3 , Tagln , and Acta2 in NCCs at E10.5 is illustrated in Fig. 3j . A subset of pharyngeal NCCs, expressing Hoxb3 that serves as a marker for PA3-6 as well as Tbx2 and Tbx3 , will form the CNCCs (cluster C2) and we refer to these cells as cardiopharyngeal NCCs (CP-NCCs; Fig. 3j ). Therefore, CNCCs can be subdivided into four populations based on position and expression of cardiac or smooth muscle genes, referred to as CP-NCCs (contained in clusters C1, C3, C5, E9.5; C2, E10.5), PAA-CNCCs of PAAs expressing Acta2, Tagln, Tbx2 , and Tbx3 (contained in C10, E10.5), OFT-CNCCs of the OFT expressing Isl1 and Gata3 (contained in Clusters C1 and C3 E9.5; C3 and C4, E10.5) and SM-CNCCs of the OFT that express Acta2 and Tagln (Clusters C14, E9.5; C10, E10.5; Fig. 3j ). We noted earlier that some CNCCs were located in clusters from PA1 and PA2 at E9.5 (C1; Fig. 2a ), that are not typically considered to harbor CNCCs. Consistent with this, at E9.5 (20 somites), we found that the OFT was connected to PA2, and CNCCs from PA2 were entering the OFT (Fig. 2g , left). At late E9.5 (24 somites), the OFT was located between PA2 and PA3, and CNCCs from PA2 and PA3 were entering the OFT (Fig. 2g , right). These data are consistent with evidence from a previous report [31] , that NCCs from anterior arches also contribute to the developing heart. Cardiac NCC fate dynamics that drive differentiation to smooth muscle cells To uncover CNCC fate dynamics at E9.5, we used CellRank software [32] (Fig. 2h, i ). We discovered genes that were progressively activated during the transition from pharyngeal NCCs to SM-CNCCs, which are candidate cardiac lineage driver genes (Fig. 2j, k and Supplementary Data 4 for the full list of genes). Our analysis indicates that CNCCs progressively activate Tbx2 , Tbx3 , Msx2, Hand2 , Gata3 , and Isl1 expression during their commitment towards SM-CNCCs at E9.5 (Fig. 2j, k ). To understand how NCCs progress at E10.5, when there are more SM-CNCCs in the pharyngeal arches, we used CellRank software and generated PAGA (partition-based graph abstract) plots (Fig. 4a–c ). The cell fate probability map from CellRank identified cells with a high potential to differentiate to smooth muscle fates (from cluster C2 and C3 to C10; Fig. 4c ). The PAGA plots further indicated that some pharyngeal NCCs (cluster C2) are CP-NCCs and they transition to OFT-CNCCs (cluster C3) that then transition to SM-CNCCs (cluster C10; blue color fraction in the pie chart; Fig. 4c ). This data also indicates that a small fraction of CP-NCCs may directly differentiate to smooth muscle cells (blue fraction in the pie chart in C2 indicates a high probability of a fraction of cells in C2 to transition directly to C10), in agreement with Tbx2 and Tbx3 expression in PAA-CNCCs at E10.5 (Fig. 3f, h, i ). We next identified genes whose expression correlates with SM-CNCC fate acquisition (Fig. 4d, e and see Supplementary Data 5 for a full list of genes at E10.5). Fig. 4: Identification of transition genes and their function at E10.5. a CellRank UMAP plot directed by RNA velocity and cell-cell similarity for clusters C2, C3, C4, and C10 from the feature plot in Fig. 3a . b UMAP plot for cell fate probabilities of CNCCs differentiating towards smooth muscle cells. c Directed PAGA plot of NCCs. Pie charts show summarized fate probabilities of individual clusters, with blue representing the proportion of cells in each cluster with high probability to become smooth muscle CNCCs of a cluster, C10. d Heatmap from CellRank showing the expression of selected genes whose expression correlates with transitions of CNCCs fate probabilities, with cells ordered by smooth muscle fate probabilities as latent time (see Supplementary Data 5 for a full list of genes), Asterisk (*) marks newly identified genes connected to CNCCs. e UMAP plots showing expression of marker genes in CNCCs. f GO enrichment analysis of four groups of genes between Bmp4 and Gata6 (defined by their pseudotime; Supplementary Data 6 ). Example of genes for each selected GO: biological processes are provided. The size of the dots indicates the adjusted p value by Bonferroni and Hochberg correction (Hypergeometric test); adjusted p value are indicated in Supplementary Data 6 . Full size image We mined the literature focusing on genes encoding transcription factors and signaling molecules, which traditionally have roles in cardiac development and modulating cell fate at E9.5 and E10.5 (Figs. 2 j, 4d ). Representative genes, with a focus on transcription factors, signaling genes, and early smooth muscle markers, were ordered according to their expression peak in pseudotime (Figs. 2 j, 4d ). While some are known to function in NCCs for heart development ( Sema3c , Msx2 , Hand1 , Hand2 , Gata4 , Gata6 , Nrp1 , Prdm6 , and Smad7 ), we found others that are newly recognized that may be required in NCCs for heart development, such as Tbx2 and Tbx3 (stars; Figs. 2 j, 4d and Supplementary Fig. 6 ). We generated lineage driver gene sets at E10.5 by dividing the genes in the fate probabilities heatmap from Bmp4 to Gata6 , least to most differentiated to SM-CNCCs, amounting to approximately 900 genes, to four groups of equal size (Supplementary Data 5 ). Next, we performed a Gene Ontology (GO) enrichment analysis of each set using ToppGene Suite [33] to understand the function of the genes in each group (Fig. 4f and Supplementary Data 6 ). Our analysis indicates that the initially activated genes of pharyngeal NCCs that include some CP-NCCs, are associated with general embryonic and mesenchyme development processes (e.g., Hox , Dlx , and Six2 genes). Then cell division (cell cycle) genes are highly expressed, consistent with the expansion of pharyngeal NCCs during development [34] , together with cardiac development genes. Finally, genes important in cardiac development and actin-filament processes ( Hand1, Gata3/4/5/6, Isl1, and Acta2 ) become strongly expressed (Fig. 4f ). In addition, our functional enrichment analysis of the fourth, most differentiated set, identified genes associated with congenital heart diseases ( Gata4/6 , Hand1/2 , Tbx20 , Nrp1 , and Acta2 ) such as tetralogy of Fallot, double outlet right ventricle and ventricular septal defects in the most differentiated cells (Supplementary Data 6 ), which supports the importance of the genetic program of CNCCs in OFT formation and disease. Furthermore, we integrated our scRNA-seq data from control embryos at E8.5, E9.5, and E10.5 and investigated the cardiac cell fate trajectory (Supplementary Fig. 7 ) using the same approach as for individual data analysis at E9.5 and E10.5. Cardiac fate trajectory analysis of the integrated data provides confirmatory information of our results from individual data analysis as progressive activation of the same specific genes during cardiac fate acquisition were found. Thus, here we identified a specific CNCC transcriptomic signature at E9.5-10.5 and revealed that cell fate acquisition to smooth muscle cells requires a multistep specification process. We additionally identified transcription factor and signaling genes such as Dkk1 , Gata3 , Foxf1 , Mef2c , Isl1 , Isl2 , Tbx2 , Tbx3 , Rgs5, Bambi , and Smad6 , among others, which have not yet been considered as CNCC transition markers (Supplementary Data 4, 5 ). Tbx2 and Tbx3 are required in cardiac NCCs for aortic arch branching Tbx2 and Tbx3 are expressed in multiple tissue types within the pharyngeal apparatus and global inactivation of both genes lead to early embryonic lethality with severe cardiac defects [35] , [36] , [37] , [38] . To understand the requirement of Tbx2 and Tbx3 in NCCs, we generated Wnt1-Cre/+;Tbx2 f/f ;Tbx3 f/f double conditional mutant embryos ( Tbx2/3 cKO). We performed intracardiac ink injection, arterial branching analysis, and histological analysis at E15.5 (Fig. 5a–l ) and found that 38.5% of Tbx2/3 cKO embryos had an aberrant retro-esophageal right subclavian artery (ARSA), 25% of Tbx2/3 cKO embryos had hypoplasia of the aortic arch but no intracardiac defects (Fig. 5a–l, m ). No defects were identified in Wnt1-Cre/+;Tbx2 f/f ;Tbx3 f/+ nor in Wnt1-Cre/+;Tbx2 f/+ ;Tbx3 f/f , in which three of four alleles were inactivated in embryos. Fig. 5: Tbx2 and Tbx3 are required together for aortic arch artery and arterial branching from the aortic arch. a – c Intracardiac ink injection of control ( a ) ( n = 3) and Wnt1-Cre;Tbx2 f/f ; Tbx3 f/f conditional null mutant embryos at E15.5 ( b , c ) ( n = 3). Panel b shows a double Tbx2/Tbx3 cKO embryo with an aberrant retro-esophageal right subclavian artery (ARSA). d – l Hematotoxin and Eosin staining on traverse sections of control ( d , f ) ( n = 18) and Tbx2/Tbx3 cKO mutant embryos ( g – l ) ( n = 9) at E15.5. Scale bars: 300 μm. Panels g and h show a Tbx2/3 cKO embryo with ARSA and panels j and k show a Tbx2/3 cKO embryo with a normal right subclavian artery. Panel i shows a Tbx2/3 cKO embryo with aortic arch hypoplasia and panel l shows a Tbx2/3 cKO embryo with a normal aortic arch as compared with control embryos ( f ). m Table of the cardiovascular defects in Tbx2/Tbx3 conditional mutants. ARSA was identified in 5/13 Tbx2/3 cKO embryos: one after intracardiac ink injection, three after H&E histology, and one by anatomic analysis after micro-dissection. Aortic arch hypoplasia was found in 2/8 Tbx2/3 cKO embryos after H&E histology. n – q Immunofluorescence on coronal sections of controls at E11.5 ( n ) ( n = 8) and Tbx2/3 cKO embryos ( o – q ) ( n = 8), at the level of the pharyngeal arch arteries for GFP and ACTA2 expression. Nuclei are stained with DAPI. Scale bars: 100 μm. The bottom panels are a high magnification of the dashed regions in n – q . Note the strong reduction of ACTA2 expression, ranging from almost total absence to low-level expression, in the right and left fourth PAAs in Tbx2/3 conditional mutant embryos compared to control embryos (white arrowheads). RSA right subclavian artery, RCC right common carotid, LCC left common carotid, BA brachiocephalic artery, Ao aorta, AoA aortic arch, LSA left subclavian artery, PT pulmonary trunk, E esophagus, PAA pharyngeal arch artery. Full size image The right subclavian artery and aortic arch are formed from the right and left 4 th PAA, respectively. By immunostaining on coronal sections of Wnt1-Cre/+;Tbx2 f/f ;Tbx3 f/f ;ROSA-EGFP f/+ embryos at E11.5 using GFP and ACTA2 antibodies, we found that NCCs contributed normally to the right and left fourth PAAs but partially or completely failed to differentiate into smooth muscle cells (Fig. 5n–q ). The failure of differentiation ranges from almost no expression of ACTA2 (Fig. 5o ) to a low level of expression (Fig. 5p, q ). This variation might explain the partial penetrance of defects in mutant embryos. We qualitatively analyzed control versus Wnt1-Cre/+;Tbx2 f/f ;Tbx3 f/f embryos at E15.5 to compare to the thickness of the muscular wall of the RSA (control and Tbx2/3 cKO without ARSA) and with ARSA (Supplementary Fig. 8 ). We found reduced thickness and reduced number of muscle layers in the ARSA of Wnt1-Cre/+;Tbx2 f/f ;Tbx3 f/f embryos, suggesting an absence of the smooth muscle layer, consequently to a possible failure of smooth muscle differentiation. Bmp4 and Foxf1 have been identified as regulators of smooth muscle cell differentiation in other organs [39] . We found that Bmp4 and Foxf1 expression was activated temporally after Tbx2 and Tbx3 expression during cardiac fate acquisition (Fig. 4d ). Disruption of cardiac NCCs by loss of Tbx1 In Tbx1 null mutant embryos, the caudal pharyngeal apparatus is hypoplastic and unsegmented at E9.5 and E10.5 due in part to the failed deployment of NCCs [9] . Further, CNCCs fail to enter the shortened cardiac OFT, leading to a persistent truncus arteriosus later in development [9] . We found that Tbx1 was not noticeably expressed in NCCs (Supplementary Fig. 9 ) and its conditional deletion in NCCs using Wnt1-Cre did not lead to cardiac defects (Supplementary Fig. 10 ). To understand how the absence of Tbx1 non-autonomously affects the development of CNCCs, we performed scRNA-seq of NCCs isolated from the microdissected pharyngeal region plus the heart of Tbx1 null mutant embryos at E9.5 (Fig. 6a ). We obtained sequencing data from 11,301 NCCs (Supplementary Table 1 ) and integrated scRNA-seq data from control and Tbx1 null embryos using RISC (Robust Integration of scRNA-seq) software [40] (Fig. 6b ). Even though there were visibly fewer NCCs in the pharyngeal apparatus (Fig. 6a ), surprisingly, there were no missing cell clusters in Tbx1 null embryos (Fig. 6b, c ). We confirmed that most of the cells in each cluster of the integrated control and Tbx1 null scRNA-seq dataset (shown in Fig. 6b ) were also clustered together in the individual datasets (Fig. 1e and Supplementary Fig. 11 ). This indicates that although affected, the general transcriptional profiles of the CNCCs are still conserved between control and Tbx1 null embryos. We then compared the proportion of cells in each cluster among the total number of NCCs in each dataset. As expected, there was a reduction in the relative proportion of NCCs in Tbx1 null embryos as compared to controls, as shown in Fig. 6 d, in PA3 (C4,1.5 fold), in proximal PA2 (C8, 1.4-fold), in early migrating NCCs in PA2 and PA3 (C9, 1.2-fold), and in early migrating NCCs in PA1 (C5, 1.4-fold). In addition, there was an increase in the relative proportion of NCCs in the distal part of PA1 and PA2 (C3; 1.6-fold; Fig. 6d ). The increase in the proportion of NCCs is consistent with previous data that cells from PA2 abnormally migrate to PA1 in Tbx1 null embryos at this stage [9] . Fig. 6: Upregulation of the BMP pathway and downregulation of the MAPK pathway by inactivation of Tbx1 at E9.5. a Wnt1-Cre;ROSA-EGFP lineage tracing (green) shows mis-localization and a reduced number of NCCs within the pharyngeal region of Tbx1 null embryos (red arrow) ( n = 10). DAPI is in blue. NCCs from the region between the two dashed lines were used for scRNA-seq. b RISC UMAP plot of integrated scRNA-seq data from NCCs of control and Tbx1 null embryos. c UMAP plots colored by clusters from control (left) and Tbx1 null embryos (right). d Stack bar graph shows proportions of NCCs in indicated clusters divided by the total number of cells in control or Tbx1 null embryos. A two-sided proportion z -test was used to evaluate cell proportion differences between control and Tbx1 null embryos (cluster C3: p value = 1.14e-56; C4: p value = 9.24e-15; C5: p value = 1.46e-8; C8: p value = 1.23e-5; C9: p value = 4.32e-3; C12: p value: 0.66) (* p value <0.05; ns not significantly different). Additional information on statistical analysis is provided in the Source Data files. e , f Scatter plots show differential gene expression in cluster C8 ( e ) and in cluster C4 ( f ) from control and Tbx1 null embryos. Note the upregulation of genes involved in the BMP pathway (red) and the downregulation of genes in the MAPK pathway (purple). g Violin plots showing differential expression in control (purple) versus Tbx1 null (red) for Msx2 , Bambi , Spry1 , and Myc in clusters C4 and C8. PA pharyngeal arch, OV otic vesicle, OFT outflow tract. Scale bars: 100 μm. Full size image Altered BMP and MAPK signaling pathways in the absence of Tbx1 We examined the data to identify differentially expressed genes (DEGs) in mutant versus control embryos at E9.5 (Supplementary Data 7 ). One of the most notable changes in Tbx1 null embryos was an increase in the expression of genes that act downstream of BMP signaling in proximal PA2 and PA3 (clusters C4, C8; Fig. 6e–g ). This includes increased expression of Msx2 , Msx1 , Bambi , Dkk1 , Smad7 , Id2 , and Id3 . Our analysis also revealed a downregulation of the expression of genes in the MAP kinase (mitogen-activated protein kinase) signaling pathway, including Spry2 , Spry4 , Myc , Foxo1 , and Lyn (Fig. 6e–g ). Signaling by BMP [41] and growth factors activating the MAPK pathway [42] , [43] are two signaling pathways known to be critical in NCCs for cardiac development. The increase in expression of Msx2 (downstream in the BMP pathway), as well as reduced expression of Spry1 (MAPK pathway) in scRNA-seq data of Tbx1 null embryos, was observed in feature plots (Fig. 7a ). We confirmed reduced MAPK signaling in pharyngeal NCCs of Tbx1 null embryos at E9.5 by performing wholemount immunostaining for P-ERK (phospho-ERK; Fig. 7b ). Expression of BMP downstream genes, Msx2 and Bambi , were expanded dorsally in Tbx1 null mutant embryos by wholemount RNAscope in situ and 3D reconstruction (Fig. 7c ). These results were confirmed by RNAscope assays on traverse sections of control and Tbx1 null embryos (Fig. 7d ). Normally, BMP signaling is most active in the ventral part of the pharyngeal apparatus near the OFT. We found an increase and ectopic expression of P-SMAD1/5/9 in the dorsal pharyngeal region, marking an increase in BMP signaling in NCCs in Tbx1 null embryos (PA2, PA3; Fig. 7e ). NCCs migrate from the dorsal to ventral parts of the pharyngeal apparatus. Our results indicate that the BMP pathway is prematurely activated during their migration in a more dorsal region of the pharyngeal apparatus compared to control embryos. These data suggest that altered BMP and MAPK signaling might affect NCC development in Tbx1 null embryos. A schematic representation of expanded and premature BMP signaling activity and reduced NCCs migrating to the shortened OFT in Tbx1 null embryos at E9.5 is shown in Fig. 7f . Fig. 7: BMP pathway is downregulated and the MAPK pathway is upregulated in pharyngeal NCCs of Tbx1 null embryos at E9.5. a UMAP plots show the expression level (purple) of Msx2 and Spry1 in NCCs split by control and Tbx1 null embryos. b Wholemount immunostaining through Wnt1-Cre;ROSA-EGFP control ( n = 7) and Tbx1 null embryos ( n = 5) for GFP (green) and phospho-ERK (pERK) (red). Digitally generated sections are shown in b . DAPI is in blue. Arrowheads show reduced expression of pERK in NCCs in the pharyngeal region of Tbx1 null embryo. c Msx2 , Bambi , and Egfp wholemount RNAscope in situ hybridization with DAPI of control and Tbx1 null embryos. ( Msx2 in control: n = 7, Msx2 in Tbx1 null embryos: n = 3, Bambi in control and Tbx1 null embryo: n = 3) The arrowheads indicate ectopic expression of Msx2 and Bambi in Tbx1 null embryos. d Egfp , Msx2 , and Bambi RNAscope assay on transverse sections of control and Tbx1 null embryos ( n = 3) showing ectopic and dorsal expression of Msx2 and Bambi in migrating NCCs (red arrowheads). Msx2 and Bambi expression is absent in the proximal part of the PA2 and PA3 of control embryos (white arrowheads). e Fluorescent immunostaining for GFP and P-SMAD1/5/9 on transverse sections of control ( n = 5) and Tbx1 null ( n = 4) embryos shows increase in P-SMAD1/5/9 in NCCs of PA2-3 (arrowheads). f Schematic representation of control (left) and Tbx1 null (right) sections at E9.5 showing reduced CNCCs contributing to the shortened OFT and ectopic posterior BMP signaling. PA pharyngeal arch, OFT outflow tract, NT neural tube, end endoderm, LV left ventricle. Scale bars: 100 μm. Full size image Cell-cell communication from the mesoderm to NCCs is disrupted in the absence of Tbx1 During the formation of the heart, NCCs receive critical signaling from adjacent mesodermal cells (Fig. 8a ). We investigated cell-cell communication and how it is disrupted in the absence of Tbx1 at single-cell resolution using CellChat software [44] . Fig. 8: Cell-cell communication from the mesoderm to NCCs is altered in the absence of Tbx1 at E9.5. a Schematic representation of a transverse section showing signaling (arrows) from pharyngeal mesoderm cells (blue) to NCCs (yellow) in the caudal pharyngeal apparatus. b Bubble plot shows representative cell-cell signaling from Mesp1 Cre derived mesodermal cells to NCCs that were significantly altered (Wilcox rank two-sided test without multiple test correction, p value indicated by the size of dot and color; right) in Tbx1 mutant embryos. Each dot represents a ligand–receptor pair interaction (Y-axis) between a specific cluster in the mesoderm cells and NCCs (X-axis). Clusters include anterior and posterior second heart fields (aSHF, pSHF) and the multilineage progenitors (MLP). c UMAP from integration of two replicates of Mesp1 Cre ; ROSA-EGFP (CTRL) and Mesp1 Cre ;Tbx1 f/f ;EGFP ( Tbx1 cKO) datasets. d UMAP plots showing Isl1 expression in control and Tbx1 cKO cells. e – m UMAP plots showing the expression of ligand genes including Wnt5a ( e ), Wnt2 ( f ), Sema3c ( g ), Pdgfa ( h ), Nrg1 ( i ), Fgf10 ( j ), Edn3 ( k ), Bmp4 ( l ), and Bmp7 ( m ) in control and Tbx1 cKO embryos. Arrows indicate cell clusters with gene expression changes in Tbx1 cKO embryos. n Wholemount RNAscope in situ hybridization of Wnt1-Cre;ROSA-EGFP control (lefts panels) and Tbx1 null (right panels) embryos at E9.5 with probes for Egfp and Bmp 4. Representative digital sections are shown on the right of 3D reconstruction pictures. Arrowheads show expression of Bmp4 in cells adjacent to the pharyngeal NCCs in Tbx1 null embryos. PA pharyngeal arch. Scale bars: 200 μm. Full size image Inactivation of Tbx1 in the mesoderm results in similar pharyngeal hypoplasia and altered NCC distribution as in global null embryos, implicating the pharyngeal mesoderm as being critical to signal to NCCs [45] . To identify Tbx1 -dependent signals from the mesoderm to NCCs, we investigated existing scRNA-seq data from Mesp1 Cre control and Tbx1 conditional null embryos at E9.5 [46] . The scRNA-seq from two replicates of Mesp1 Cre control and Tbx1 conditional null embryos were integrated using RISC software as described [46] . We focused on mesodermal subpopulations, expressing Tbx1 , that are adjacent to the NCCs, including the anterior and posterior second heart field (aSHF; pSHF) [47] , [48] . We also included a critical Tbx1 -dependent multilineage progenitor population (MLP) in the pharyngeal mesoderm required for cell fate progression to the aSHF and pSHF [46] . We examined signaling to NCCs in clusters corresponding to migrating NCCs of the future PA2-3 (C9), distal part of PA1-2 (C3), mesenchyme of PA2 (C8) and PA3 (C4), and CNCCs of the OFT (C12) in integrated scRNA-seq data from control and Tbx1 null embryos at E9.5 (Figs. 6 , 8b ). Representative results of ligand–receptor pairs altered when Tbx1 is inactivated are shown in Fig. 8b , and the complete set of pairs are in Supplementary Fig. 12 . Affected ligands in the mesoderm include Wnt5a, Wnt2, Sema3c, Pdgfa Nrg1, Fgf8, Fgf10, Bmp4 , and Edn3 and others. To validate relationships, we analyzed integrated Mesp1 Cre data (Fig. 8c ; MLPs-C8, aSHF-C10, and pSHF-C1 + C12). Isl1 , is a critical gene required for OFT development [49] , and it is expressed in the MLPs, aSHF, and pSHF (Fig. 8d ). We examined expression changes in feature plots of Wnt5a , Wnt2 , Sema3c , Pdgfa , Nrg1 , Fgf10 , and Edn3 as well as other genes (Fig. 8e–m ). These genes were altered in expression in the cell types specified and, in the direction of altered signaling (decreased or increased in the mutant embryos), as indicated in Fig. 8b . Reduced expression of Wnt5a [50] , [51] , Fgf8 [46] , [52] , [53] , Fgf10 [54] , [55] , Sema3c [56] , and Nrg1 [46] ligands and increase of Wnt2 [57] are consistent with previous in vivo studies of Tbx1 mutant embryos; however, these were not known with respect to cell-cell communication to NCCs. With these data, we show, on a single-cell level, that signaling to NCCs is altered in Tbx1 mutant embryos. We also identified ligand–receptor pairs that were not previously connected to NCCs or Tbx1 . Two ligand genes, Edn3 and Pdgfa were identified in our cell-cell communication analysis (Figs. 8 h, k ). Edn3 encodes an endothelin ligand important in cell migration. Pdgfa encodes a growth factor regulating cell survival, proliferation, and migration and PDGF signaling is required in NCC development [58] . To our knowledge, there is no report of Edn3 and Pdgfa having been investigated in relation to Tbx1 . We investigated CellChat results for the BMP and MAPK pathways that were altered in NCCs when Tbx1 was inactivated. An abnormal increase of the BMP signaling from the mesoderm to NCCs in Tbx1 mutant embryos was found through Bmp4/5/7 ligands (Fig. 8b ). We performed RNAscope in situ hybridization for expression of Bmp4 and Bmp7 (Fig. 8n and Supplementary Fig. 13 ). Bmp4 is expressed in the pharyngeal mesoderm and Bmp7 is expressed in the pharyngeal mesoderm and endoderm adjacent to the NCCs. Expression of these two ligands were maintained in Tbx1 null embryos as compared to control embryos at E9.5 (Supplementary Fig. 13 and Fig. 8l, m ). Fgf8 and Fgf10 are ligands in FGF signaling that act through the MAPK pathway and it is well known that they are reduced in expression in Tbx1 mutant embryos [46] , [52] , [53] , [54] , [55] (Fig. 8j ). Similarly, we found that Fgf8 and Fgf10 were reduced in expression in the mesoderm and signaling to NCCs was altered (Fig. 8b ). It is known that FGF signals to NCCs during embryonic development [42] , [59] , [60] . Therefore, it is possible that the reduction of FGF and/or increase in BMP, along with changes in other ligands in the adjacent mesoderm, could lead to their failed progression and cardiac contribution. Failed cardiac cell fate progression of NCCs in the absence of Tbx1 at E10.5 To further understand how the contribution of NCCs to the OFT is altered in the absence of Tbx1 , we performed scRNA-seq of NCCs in Tbx1 null embryos at E10.5, when the caudal pharyngeal apparatus is hypoplastic (Fig. 9a ). We integrated scRNA-seq data from two control replicates (21,561 cells) and two Tbx1 null replicates (17,840 cells) using RISC software (Fig. 9b ). We confirmed that most of the cells in each cluster of the integrated control and Tbx1 null scRNA-seq dataset (shown in Fig. 9b ) were also clustered together in the individual datasets (Fig. 1f and Supplementary Fig. 14 ). The integrated datasets clearly show a strong reduction in the number of NCCs in most clusters in Tbx1 null embryos including OFT-CNCCs ( Isl1/Gata3 +; C10) and SM-CNCCs ( Acta2 +; C13) as shown in Fig. 9c , except that the relative proportion of pharyngeal NCCs that contain CP-NCCs ( Tbx2/Tbx3 +; C4) was not significantly changed, after considering the total cells being sequenced (Fig. 9d ). Fig. 9: Failure of CNCC cell fate progression by loss of Tbx1 at E10.5. a The NCCs between the dotted lines and heart in control and Tbx1 null embryos were used for scRNA-seq. b RISC UMAP plot of integrated scRNA-seq data from NCCs of two replicates of control and Tbx1 null embryos. c UMAP plots of pharyngeal and heart clusters from control (left) and Tbx1 null (right) embryos. d Stack bar graph shows proportions of NCCs in selected clusters divided by the total cell number in control or Tbx1 null replicates. A two-sided proportion z -test was used to evaluate cell proportion differences between control and Tbx1 null embryos for the two replicates separately if the two Tbx1 null show consistent increase or decrease compared to control. (* p value <0.05; ns not significantly different, see Source Data file for p value details). e UMAP plot colored by cell fate probabilities. f UMAP plots showing expression level of Tbx2 , Tbx3 , Isl1, Gata3 , Msx2 , and Dkk1 in NCCs from control or Tbx1 null embryos in pharyngeal NCC clusters. Msx2 , Gata3 , and Dkk1 show increased expression in cluster C4. g Violin plots showing differential expression level of Msx2 , Bambi , Gata 3, and Tbx2 in cluster C4 in control (purple) and Tbx1 null (red) embryos. h – j GO analysis for upregulated genes in C4 ( h ), downregulated genes in C4 ( i ), and upregulated genes in C10 ( j ). Hypergeometric test was used, adjusted p value by Bonferroni–Hochberg correction. k Fluorescent immunostaining for GFP (green) and ISL1 (red) with DAPI (blue) on transverse sections of control ( n = 4) and Tbx1 null ( n = 3) embryos. There is reduced ISL1-positive NCCs (arrowheads). l Fluorescent immunostaining for GFP (green), TBX2 (red), and ACTA2 (gray) on transverse sections of control ( n = 4) and Tbx1 null ( n = 3) embryos, DAPI is in blue. Expression of TBX2 in NCCs is lateral to the pharyngeal endoderm (end; white arrowheads). There are fewer CNCCs expressing ACTA2 within the OFT of Tbx1 null embryos (red arrowhead). NT neural tube, end endoderm, OFT outflow tract. Scale bars: 100 μm. Full size image Our analysis showed that the cell fate probabilities point from pharyngeal NCCs containing CP-NCCs (C4) and OFT-CNCCs (C10) toward SM-CNCCs (C13) as shown in Fig. 9e . We generated a list of DEGs in clusters C4 and C10, between control and mutant embryos at E10.5 (Supplementary Data 8 ). Msx2 , Bambi , Gata3 , and Dkk1 were increased and abnormally expressed in pharyngeal NCCs (cluster C4) in Tbx1 null embryos (Fig. 9f, g and Supplementary Data 8 ). This suggests that an abnormal upregulation of BMP signaling occurred in the absence of Tbx1 , consistent with data at E9.5 in Fig. 8 . GO analysis of the upregulated genes in pharyngeal NCCs (cluster C4) confirms the upregulation of BMP signaling in Tbx1 null embryos (Fig. 9h and Supplementary Data 9 ). By GO analysis, we found downregulation in the expression of genes involved in embryonic organ development and mesenchyme development in pharyngeal NCCs that contain CP-NCCs (Fig. 9i and Supplementary Data 10 ), suggesting dysregulation of NCC development. We also noted that there was an upregulation of genes that inhibit the cell cycle progression of OFT-CNCCs (Fig. 9j and Supplementary Data 11 ). By immunostaining, we confirmed the overall reduction in the number of CNCCs within the OFT and NCCs in the pharyngeal region of Tbx1 null embryos (Fig. 9k, l ). We also confirmed a reduced number of ISL1 + NCCs in the dorsal aortic sac wall mesenchyme and distal OFT, as well as the absence of the aortic sac protrusion in Tbx1 null embryos (Fig. 9k ). Supporting the scRNA-seq data, immunostaining experiments indicated that TBX2 (and likely TBX3) expression was maintained in NCCs located in the lateral part of the pharyngeal apparatus (Fig. 9l ). 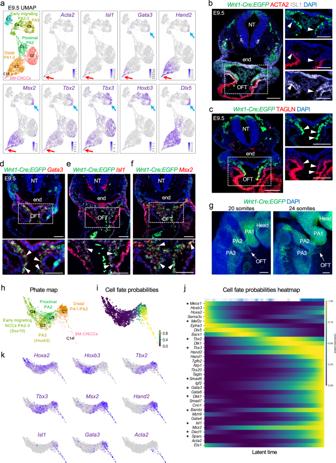Fig. 2: Transcriptional dynamics of cardiac NCCs at E9.5. aUMAP plots of scRNA-seq data with genes that mark CNCCs identified by expression ofActa2,Isl1,Gata3,Hand2,Msx2,Tbx2, andTbx3with respect toHoxb3(PA3) andDlx5(distal PA1, 2, 3) expression (red arrows). Blue arrows show the expression ofGata3,Hand2,Msx2,Tbx2, andTbx3in the distal part of PA3.b,cImmunostaining on traverse sections throughWnt1-Cre;ROSA-EGFPembryos showingCre-activated EGFP (green), ACTA2, TAGLN, and ISL1 protein expression. Nuclei (blue) are labeled with DAPI. White arrowheads indicate CNCCs expressing ACTA2 and ISL1 (n= 3) (b) and CNCCs expressing TAGLN (n= 3) (c) in the OFT.d–fRNAscope analysis ofWnt1-Cre;ROSA-EGFPembryos forEgfp,Gata3(d) (n= 3),Isl1(e) (n= 3), andMsx2(f) (n= 4) expression. Nuclei (blue) are labeled with DAPI. Arrowheads indicate the expression ofGata3,Isl1, andMsx2in CNCCs within the OFT.gWholemount RNAscope analysis ofWnt1-Cre;ROSA-EGFPembryos at 20 and 24 somites where the position of the OFT is indicated (white arrowhead).hPHATE (potential of heat-diffusion for affinity-based transition embedding) map of NCCs in clusters C1, C3, C4, C5, and C14 using Louvain clustering.iPHATE map colored by cell fate probabilities, showing how each cell is likely to transition to SM-CNCCs as defined by CellRank software (yellow represents high cell fate probabilities).jHeatmap from CellRank showing the expression of marker genes whose expression correlates with cardiac fate probabilities as latent time, with cells order by fate probabilities as latent time (see Supplementary Data4for a full list of genes), Asterisk (*) indicates newly identified genes connected to CNCCs.kPHATE maps with an expression of marker genes of CNCCs at different states of differentiation towards smooth muscleActa2expressing cells. NT neural tube, end endoderm, OFT outflow tract, PA pharyngeal. Scale bars: 100 μm. We also noticed that there was normal differentiation of the CNCCs within the OFT of Tbx1 null embryos despite that there are fewer cells (Fig. 9l ). Together this suggests a reduction but not a complete failure of cardiac fate progression between pharyngeal NCCs and OFT-CNCCs states in the absence of Tbx1 . In this report, we identified the cell type signatures and cell fate dynamics of CNCCs. We focused on pharyngeal NCCs in the mouse at developmental stages when Tbx1 , the gene for 22q11.2DS, is highly expressed and functions. We determined the mechanisms by which Tbx1 non-autonomously regulates CNCC maturation at a single-cell level and found that altered BMP and FGF-MAPK signaling, together with other signaling, may contribute to cardiovascular malformations when Tbx1 is inactivated. We also uncovered genes and ligand–receptor pairs with respect to cell-cell communication from mesoderm to NCCs that add to our understanding of CNCC fate progression. NCCs are multipotent and differentiate into many cell types, including smooth muscle cells. Through examination of transitional dynamics along with embryonic localization by in situ analysis, we uncovered three main transition states from pharyngeal to smooth muscle expressing CNCC derivatives, termed CP-NCCs, OFT-CNCCs, and SM-CNCCs as shown in the model in Fig. 10a . Fig. 10: Model of a multistep specification to form CNCCs and the signaling pathways disrupted by inactivation of Tbx1 . a Colors indicate cell fate progression of pharyngeal NCCs (light yellow) towards vascular smooth muscle cells (red). Step 1 shows the transition between pharyngeal NCCs expressing Tbx2/3 to cells expressing markers of CNCCs (CP-CNCCs). Step 2 shows the transition in which some cells directly differentiate to smooth muscle of PAA-CNCCs, while the majority migrate and enter the OFT as OFT-CNCCs and express Gata3/Isl1 and Step 3 shows the transition to SM-CNCCs expressing Acta2 . The graph shows the relative change of biological gene ontology terms during the three transitions of CNCCs to smooth muscle cells. b Model of non-autonomous signaling between the mesoderm (bottom, blue) and NCCs (top, gray) highlighting FGF, WNT, and additional signaling from the mesoderm to NCCs in normal embryos (left) and how signaling is disrupted in the absence of Tbx1 (light blue arrows/inhibitory arrows; right). Alteration of signaling in the mesoderm in the absence of Tbx1 results in abnormal premature activation of the BMP pathway during NCC deployment and migration (light blue inhibitory arrow; red, up arrow), a decrease of MAPK signaling in NCCs (light blue arrow; red down arrow), and alteration of other signaling pathways including upregulation of WNT signaling in developing NCCs. This leads to failure of cardiac fate progression with a reduced number of CP-CNCCs, reduced number of CNCCs, and reduced number of SM-CNCCs (gray arrows) with aortic arch/branching defects and failed OFT septation (persistent truncus arteriosus). Full size image The CP-NCCs express Hox and Dlx genes, as well as those implicated in cardiac development, including Tbx2 and Tbx3 , as well as other genes (Fig. 10a ). Our data also suggests that some Tbx2/3 + cells differentiate directly into Acta2 + smooth muscle cells in the PAAs (PAA-CNCCs; Fig. 10a ). A role of Tbx2 and Tbx3 in CNCCs in PAA development have not been previously described, and we found that inactivation results in the partially penetrant abnormal aortic arch and arterial branching, indicating besides function as markers of CP-NCCs, they have a role in smooth muscle differentiation. Partially penetrant hypoplasia of the aortic arch and arterial branching defects of Wnt1-Cre;Tbx2 f/f ;Tbx3 f/f embryos can result from the ability of the PAAs to recover during development [13] , [61] , [62] , [63] , [64] , [65] . Another reason for partial penetrance in mutant embryos could be because mice with a mixed genetic background were used in this study. The OFT-CNCCs express cardiac transcription factors such as Hand1/2, Msx1/2, Foxf1 , and Gata3 , as well as Isl1/2 (Fig. 10a ). These cells are required for OFT development, as determined by conditional inactivation studies in NCCs of Hand2 [66] , Msx1 , and Msx2 [67] . Expression of Isl1 in CNCCs contributing to the OFT is consistent with a dual lineage tracing study [68] . We also identified genes not previously connected to CNCCs that include Dkk1 , Foxf1 , Rgs5 , Isl2 , and Gata3 , as well as newly recognized genes for cardiovascular development. SM-CNCCs are NCCs within the OFT that expresses Acta2 and Tagln smooth muscle genes together with Gata4/5/6 , Cnn1 , Tbx20 , and Smad6/7 . Supporting their requirement, conditional deletion of Gata6 in NCCs results in septation defects of the OFT [69] . Abnormal activation of Smad7 in the NCCs derived from Wnt1-Cre genetic lineage leads to pharyngeal arch and cardiac OFT defects [70] . We additionally found genes not yet connected to these cells, including Meox1 , Bambi , and Smad6 . We found that the progression of CNCC fate toward smooth muscle of the OFT is associated with progressive downregulation of genes involved in pharyngeal embryonic development and progressive increase in cardiac specification genes, consistent with maturation of the unipotent cellular state to smooth muscle cells (Fig. 10a ). Development of NCCs in the pharyngeal apparatus is regulated by cell-cell signaling, in part from the pharyngeal mesoderm, as uncovered by studies of Tbx1 mutant embryos [45] , [71] . In global null or Mesp1 Cre mediated Tbx1 conditional null embryos, there is altered deployment of CNCCs and reduced contribution to the OFT, leading to a persistent truncus arteriosus [45] , [71] . Our results suggest that NCCs are produced normally in the neural tube in the absence of Tbx1 , but they fail to migrate to the caudal pharyngeal arches and OFT, as well as to fail to progress to more mature states, as shown in our model in Fig. 10b . We suggest that failure to migrate and progress in development is due in part to disrupted signaling from adjacent mesodermal cells to the NCCs as shown in Fig. 10b . Here, we identified several receptor-ligand interactions that are disrupted by comparing scRNA-seq data from NCCs and the Mesp1 Cre lineages. Using CellChat software [44] , we identified signaling interactions from the mesoderm to NCCs and their disruption in Tbx1 mutant embryos, at a single-cell level. We identified a reduction of FGF ligand expression ( Fgf8 and Fgf10 ) in the mesoderm with reduced MAPK signaling in NCCs, as shown in the model in Fig. 10b . This confirms previous studies showing that inactivation of Tbx1 results in reduced expression of Fgf8 and Fgf10 ligands in the mesoderm [55] , [72] . It is known that loss of FGF ligands indirectly results in NCC mediated cardiovascular anomalies [42] , [59] , [60] . This function is affected significantly by the MAPK signaling pathway that is critical for NCC development and migration [42] . Further, FGF signaling is required downstream of Tbx1 , both genetically and mechanistically [52] , [54] . Reduced phospho-ERK1/2 has previously been reported in pharyngeal NCCs of Tbx1 hypomorphic embryos [73] . Finally, our bioinformatic analysis shows a reduction of downstream effector genes in the MAPK pathway ( Myc, Spry1, and Spry2 ). When taken together, our results support an essential role of mesodermal TBX1-FGF signaling to NCCs that is required for normal heart development (Fig. 10b ). We also found an increase and premature activation of BMP signaling in pharyngeal NCCs of Tbx1 null embryos along with the expansion of p-SMAD1/5/9 and downstream effector genes, Msx1/2 and others (Fig. 10b ). Inactivation of a BMP antagonist gene, Dullard in NCCs resulted in similar cardiac OFT defects as in Tbx1 null mutant embryos [41] implicating a mechanistic connection between an increase in BMP signaling and OFT defects. The CellChat analysis showed that there is an increase of Bmp4 and Bmp7 expression in the adjacent mesoderm relative to the expression of specific Bmp receptor genes. Although our RNAscope analysis of Bmp4 and Bmp7 did not show an obvious increase in the expression of these two ligands, they continue to be strongly expressed in the mesoderm of Tbx1 null mutant embryos suggesting that the source of BMP ligands is in adjacent cells that interact with NCCs. It is known that BMP4 can activate BMP signaling through p-SMAD1/5/9 [74] , [75] and this is consistent with our findings (Fig. 10b ). In the future, utilization of organoids and cell culture systems will help dissect the mechanism of how BMP interacts with NCCs. Based upon this analysis, we propose that the inactivation of Tbx1 results in an alteration of paracrine signaling from the mesoderm, including FGF and BMP, separately contributes to CNCC migration and fate progression, as shown in Fig. 10b . However, these are not the only signaling pathways that are affected by inactivation of Tbx1 . We found an increase in Wnt2 expression in the mesoderm by CellChat analysis. We previously found that global Tbx1 inactivation [76] or inactivation in the aSHF using Mef2c-AHF-Cre , resulted in increased Wnt2 expression [57] . Therefore, canonical WNT signaling also functions downstream of Tbx1 , and this may also affect NCC function. The CellChat analysis also revealed downregulation of Nrg1-Erbb3 , implicating altered Neuregulin to ERBB3 signaling in CNCCs in Tbx1 mutant embryos. Neuregulin is important for the migration of NCCs, acting as a chemoattractant and chemokinetic molecule [77] and it is involved in heart development. It has been shown recently that Nrg1 is a direct transcriptional target gene of TBX1 in the multilineage progenitors (MLPs) in the mesoderm [46] . Therefore, alteration of Neuregulin signaling in Tbx1 mutant embryos could, in part, explain the failed cardiac contribution of the NCCs. There was other signaling affected, some of which has not been investigated with respect to Tbx1 or mesoderm-NCC signaling, such as identified by alteration in expression of Edn3 or Pdgf a genes, which can be pursued in the future. Together, our analyses indicate that a combination of important signaling from the pharyngeal mesoderm to NCCs are affected in Tbx1 mutant embryos and could contribute to the failure of fate progression of CNCCs. One of the reasons for the disruption of NCCs in Tbx1 mutant embryos is failed segmentation of the caudal pharyngeal arches by the endoderm. Alternatively, disruption of NCCs could affect the pharyngeal endoderm resulting in failed segmentation. A previous study by Veitch and colleagues showed that after the ablation of NCCs in the chick embryo, pharyngeal segmentation still took place [78] . This suggests that pharyngeal segmentation defects in Tbx1 null embryos is not due to a reduced number of defective NCCs. There are many reasons for failed segmentation of the caudal pharyngeal apparatus due to Tbx1 inactivation. The tissue-specific functions of Tbx1 in this process has been evaluated. Loss of Tbx1 in the pharyngeal endoderm autonomously affects segmentation of the caudal pharyngeal apparatus leading to reduced contribution of CNCCs [79] . The pharyngeal endoderm is also an important source of signaling during development, including FGF ligands [59] , that could potentially affect NCCs development. It was found that Tbx1 expression in the mesoderm is necessary, non-autonomously, for pharyngeal segmentation [45] , suggesting that defects in signaling from the adjacent mesoderm that expresses Tbx1 , cause failed segmentation. Loss of Tbx1 in the mesoderm also leads to failed CNCC migration and fate progression. The Tbx1 expression domain in the pharyngeal ectoderm also serves as a signaling center for non-autonomous signaling [64] , [80] . It will be interesting to evaluate how the exchange of signaling between the pharyngeal epithelia and NCCs are affected in the absence of Tbx1 . In conclusion, in this report, we identified the transcriptional signature that defines the CNCCs and identified the gene expression dynamics that regulate CNCC fate progression into the smooth muscle of the OFT and PAAs. In addition, we highlight the direct alteration of FGF, BMP, and other signaling from the mesoderm to NCCs, most likely leading to failed OFT septation in the absence of Tbx1 at a single-cell level. Together our results allow a better understanding of the normal development of CNCCs and provide insights into the origin of congenital heart defects associated with defective NCCs and 22q11.2DS. Mouse lines Animal experiments were carried out in agreement with the National Institutes of Health and the Institute for Animal Studies, Albert Einstein College of Medicine ( https://www.einsteinmed.org/administration/animal-studies/ ) regulations. The IACUC protocol number is #00001034. The following transgenic mouse lines were used: Wnt1-Cre [17] , ROSA26R-GFP f/+ [18] , that we refer to as ROSA-EGFP , Tbx1 +/- [81] , Tbx1 f/+ [81] . Mice were maintained on a mixed Swiss-Webster genetic background. Tbx2 f/+ and Tbx3 f/+ mutant mouse lines were generated in Dr. Chenleng Cai’s laboratory by inserting a two LoxP site into the intron sequences flanking exon 2 of the Tbx2 gene and exons 2–4 of Tbx3 gene, by gene targeting using homologous recombination. After recombination of the genomic sequences between the LoxP sites, the reading frame and T-Box domain of Tbx2 and Tbx3 are both disrupted [82] . Tbx2 f/+ and Tbx3 f/+ mice were maintained on a mixed Swiss-Webster and C57BL/6 genetic background. Embryos were not evaluated for sex, because we studied developmental processes prior to sexual development. Mice and embryos resulting from the different crosses were genotyped from DNA extracted from the tips of toes or yolk sacs. The individual PCR primers and assays used in the experiments are described in the reports on individual mouse alleles. Embryos were collected at different embryonic days dated from the day of the vaginal plug (E0.5). For each experiment, a representative result was presented from at least three analyzed embryos. Immunofluorescence staining on paraffin sections Embryos were collected in cold 1x PBS (Phosphate Buffered Saline) and fixed in 4% PFA (Paraformaldehyde) for 1 h at 4 °C under constant agitation. Embryos were progressively dehydrated in ethanol, then xylene, and embedded in paraffin (Paraplast X-tra, Sigma P3808). The embryos were sectioned to the 10-μm thickness and sections were deparaffinized in xylene and progressively rehydrated in an ethanol series. Sections were incubated and boiled in antigen unmasking solution (Vector laboratories, H-3300) for 15 min. After cooling at room temperature, sections were washed in PBS containing 0.05% Tween (PBST) and blocked for 1 h in TNB buffer (0.1 M Tris-HCl, pH 7.5, 0.15 M NaCl, 0.5% Blocking reagent [PerkinElmer FP1020]) at room temperature. Then sections were incubated with primary antibodies diluted in TNB overnight at 4 °C. Sections were washed in PBST and incubated with secondary antibodies diluted in TNB for 1 h at room temperature. After washes in PBST, nuclei were stained with DAPI (1/1,000; Thermo Scientific, 62248) and slides were mounted in Fluoromount (Southern Biotech). Embryonic sections were imaged using a Zeiss Axio Imager M2 microscope with ApoTome.2 module. Images were analyzed using Zen software from Zeiss, ImageJ, and Adobe Photoshop. Immunofluorescence on wholemount embryos Embryos were collected in 1x PBS and fixed in 4% PFA overnight at 4 °C under constant agitation. Then embryos were washed in 1x PBS and progressively dehydrated in a methanol bath series (25, 50, and 100%) and stored at −20 °C. After progressive rehydration in 1x PBS, embryos were incubated in 1x PBS containing 0.1% Triton (PBS-Triton) overnight at 4 °C. Embryos were then incubated in blocking solution (1x PBS containing 10% Donkey serum (Sigma, D9663)) overnight at 4 °C under continuous agitation. Then embryos were incubated with primary antibodies diluted in blocking solution for 2 days at 4 °C under constant agitation. After 5 watches (1 h each) in 0.1% PBS-Triton at 4 °C, embryos were incubated with secondary antibodies, and DAPI diluted in a blocking solution for 2 days at 4 °C. Embryos were washed in 0.1% PBS-Triton five times, then progressively dehydrated in 100% methanol and cleared in benzyl alcohol-benzyl benzoate (2:1 volume per volume ratio) (BABB) solution. Embryos were imaged as a Z-stack using a Nikon CSU-W1 spinning disk confocal microscope. Images were analyzed using ImarisViewer 9.8.0 software. Antibodies used for immunostaining experiments The following primary antibodies were used: goat anti-GFP (1/200, Abcam ab6673), mouse anti-alpha smooth muscle actin ACTA2) (1/200, Abcam ab7817), rabbit anti-αSMA (ACTA2; 1/200, Abcam ab5694), mouse anti-Isl1/2 (1/100, DSHB 40.2D6 and DSHB 39.4D5), mouse anti-TBX2 (1/100, Santa Cruz sc514291), rabbit anti-TAGLN (1/200, Abcam ab14106), rabbit anti-p-SMAD1/5/9 (1/100, Cell Signaling D5B10 #13820), rabbit anti-TBX1 (1/100, Lifescience LS-C31179), rabbit anti-pERK (1/100, Cell Signaling p44/42 MAPK, 9101), and MF20 (1/100, Sarcomeric Myosin heavy chain antibody, mouse, DSHB). The following secondary antibodies were used from Invitrogen (Thermo Fisher Scientific) raised in donkey at 1/200: anti-goat IgG Alexa Fluor 488 (A11055), anti-mouse IgG Alexa Fluor 555 (A31570), anti-mouse IgG Alexa Fluor 647 (A3157), anti-rabbit IgG Alex Fluor 555 (A31572), anti-rabbit IgG Alex Fluor 568 (A10042) and anti-rabbit IgG Alex Fluor 647 (A31573). RNAscope RNAscope on wholemount embryos Embryos were collected and dissected in 1x PBS at 4 °C and fixed in 4% PFA overnight. Then embryos were dehydrated in progressive methanol washes and stored in 100% methanol at −20 °C. Wholemount RNAscope was performed using RNAscope Multiplex Fluorescent Detection Reagents v2 kit (Advanced Cell Diagnostics, ref 323110). Embryos were progressively rehydrated in 1x PBS containing 0.01% Tween (PBST) and were permeabilized using Protease III (Advanced Cell Diagnostics, ref 323110) for 20 minutes at room temperature, followed by washes in PBST. Embryos were then incubated with 100 μl of pre-warmed mixed C1, C2, and C3 (ratio 50:1:1, respectively) RNAscope probes at 40 °C, overnight. After three washes in 0.2x SSC (Saline Sodium Citrate), 0.01%Tween, embryos were fixed in 4% PFA for 10 min at room temperature. Embryos were then incubated in Amp1 for 30 min at 40 °C, Amp2 for 30 min at 40 °C, and Amp3 for 15 min at 40 °C, with washes in 0.2x SSC, 0.01%Tween between each step. Tyramide signal amplification (TSA) solutions were prepared as follows: 1/500 for TSA-Fluorescein (Akoya Biosciences, NEL741001KT), 1/2000 for TSA-CY3 (Akoya Biosciences, NEL744001KT), and 1/1,000 for TSA-CY5 (Akoya Biosciences, NEL745001KT). To reveal C1 probes, embryos were incubated in HRP1-C1 for 15 min at 40 °C, then washed and incubated with the chosen TSA solution, for 30 min at 40 °C. The amplification reaction was blocked using HRP-Blocker for 15 min at 40 °C. C2 and C3 probes were revealed following the previous steps and using HRP-C2 for C2 probes and HRP-C3 for C3 probes. Nuclei were stained overnight with DAPI. Wholemount embryos were imaged as Z-stacks using a Leica SP5 confocal microscope or a Nikon CSU-W1 spinning disk confocal microscope, after being cleared with BABB or not. 3D image reconstruction and analyses were performed using ImageJ and ImarisViewer 9.8.0 software. RNAscope on cryosections Embryos were collected and dissected in 1x PBS at 4 °C then fixed in PFA 4% overnight and incubated in successive 10, 20, and 30% sucrose (Sigma-Aldrich S8501) solutions and then embedded in OCT (Optimal Cutting Temperature compound). Embryos were stored at −80 °C until they are used. 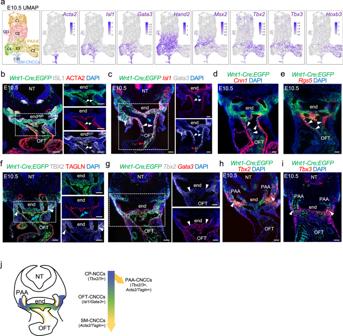Fig. 3: Transcriptional dynamics of cardiac NCCs at E10.5. aSeurat UMAP plots of scRNA-seq data from NCC populations with the expression of marker genes.bImmunostaining on traverse sections ofWnt1-Cre;ROSA-EGFPembryos (n= 3) showing GFP, ISL1, and ACTA2 expression. Nuclei stained with DAPI are in blue. ISL1 is expressed in smooth muscle cells of the OFT cushions (arrowheads).c–eRNAscope in situ hybridization sections ofWnt1-Cre;ROSA-EGFPembryos forEgfp,Isl1andGata3 (c) (n= 5),Egfp,Cnn1(d) (n= 3),EgfpandRgs5(e) (n= 3) expression. Nuclei stained with DAPI are in blue.Isl1andGata3are expressed in NCCs within the OFT (white arrowheads inc) and at the level of the dorsal aortic sac wall and aortic sac protrusion (blue arrowheads inc).Gata3but notIsl1is expressed in the more proximal part of OFT (red arrowheads inc).Cnn1andRgs5are expressed in smooth muscle cells of the OFT (white arrowheads indande).fImmunostaining on sections ofWnt1-Cre;ROSA-EGFPembryos (n= 3) showing GFP, TBX2, and TAGLN expression. Expression of TAGLN is in smooth muscle cells of the OFT (blue arrowheads) and PAAs expressing TBX2 (white arrowheads).g–iRNAscope in situ hybridization on traverse sections ofWnt1-Cre;ROSA-EGFPembryos forEgfp,Tbx2(n= 5) andGata3(n= 4) (g),EgfpandTbx2(h) (n= 5), andEgfpandTbx3(i) (n= 5) expression. Nuclei stained with DAPI are in blue.Tbx2andGata3expression overlaps in the dorsal wall of the OFT (white arrowheads ing).Tbx2andTbx3are expressed in the mesenchyme dorsal to the aorta surrounding the PAAs at the level of the PA3-6 (white arrowheads inhandi).jSchematic representation of a transverse section at the level of the OFT summarizingTbx2,Tbx3,Isl1,Gata3,Acta2, andTaglnexpression in CNCCs at E10.5. NT neural tube, end endoderm, PAA pharyngeal arch artery. Scale bars: 100 μm. RNAscope was performed on 10-μm sections mounted on SuperFrost Plus slides (Fisher Scientific, 12-550-15) following the RNAscope Multiplex Fluorescent Reagent Kit v2 assay protocol from Advanced Cell Diagnostics. Sections were imaged using a Zeiss Axio Imager M2 microscope with ApoTome.2 module. Acquisitions were processed using Zen software from Zeiss, ImageJ, and Adobe Photoshop. Probes used for RNAscope: Egfp (400281, 400281-C3), Tbx2 (448991), Hoxb3 (515851), Dlx2 (555951), Bambi (523071), Hoxa2 (451261), Gata3 (4033321-C2), Isl1 (451931, 451931-C2), Tbx3 (832891-C2), Sox10 (435931-C2), Msx2 (421851-C2), Meox1 (530641-C2), Dlx5 (478151-C3), Twist1 (414701), Rgs5 (430181-C3), Cnn1 (483791), Bmp4 (401301), and Bmp7 (407901). Histology and staining with Hematoxylin & Eosin Fetuses were collected and dissected in 1x PBS and fixed overnight in 4% PFA. They were progressively dehydrated in ethanol and incubated in xylene prior to embedding in paraffin. Tissue sections of 12-μm thickness were deparaffinized in xylene and progressively rehydrated in ethanol washes and incubated for 10 min in Hematoxylin (Sigma-Aldrich, HHS16) then rinsed in water and dehydrated in 70% ethanol. Sections were then incubated in alcoholic Eosin (70%) (Sigma-Aldrich, HT110116) solution and progressively dehydrated in ethanol and xylene washes prior to mounting in Permount mounting medium (Fisher Chemical SP15100). Sections were imaged using a Zeiss Axioskop 2 plus microscope and analyzed using Zen software and Adobe Photoshop software. Intracardiac India ink injection Fetuses at E15.5 were dissected in 1x PBS and the chest was carefully opened to avoid damaging the cardiovascular system. A solution containing 50% India ink and 50% 1x PBS was injected into the left ventricle of the heart by blowing gently into an aspirator tube assembly connected to a microcapillary. Immediately after filling the left ventricle and arterial branches, the heart and aortic arch with arterial branches were imaged using a Leica MZ125 stereomicroscope. Images were analyzed using Zen software and Adobe Photoshop software. scRNA-seq data generation Embryos were collected and microdissected in 1x PBS at 4 °C. Dissected tissues of interest were maintained in DMEM (Dulbecco’s Modified Eagle Medium, GIBCO 11885084) at 4 °C. For E8.5 embryos, the rostral half of the embryos, including the heart, was collected. The head of the embryo was conserved at E8.5 because of the small size of the embryos that most likely contain CNCC progenitors in the anterior part of the pharyngeal region. At E9.5, the pharyngeal region from PA1 onwards, plus the heart, were collected. The head of the embryos containing NCCs not relevant to the cardiovascular system were removed at E9.5 to not dilute out the pharyngeal NCCs, including CNCCs. At E10.5, the pharyngeal region plus the heart were collected. The head and PA1 were removed at E10.5, as shown in Fig. 1 , because, at this time point, these NCCs are destined to form the craniofacial skeleton, not the cardiovascular system. Then, tissues were incubated in 1 ml of 0.25% Trypsin-EDTA (GIBCO, 25200056) containing 50 U/ml of DNase I (Millipore, 260913-10MU), at room temperature for 7 min. Next, heat-inactivated FBS (fetal bovine serum, ATCC, 30-2021) was added to stop the reaction at a final concentration of 10%, at 4 °C. Dissociated cells were centrifugated for 5 min at 300 × g at 4 °C and the supernatant was removed. Cells were then resuspended in 1x PBS without Ca 2+ and Mg 2+ (Coming, 21-031-cv) containing 10% FBS at 4 °C and filtered with a 100-μm cell strainer. A total of 1 μl DAPI (1 mM) (Thermo Fisher Scientific, D3571) was added. Cells were FACS (Fluorescence Activated Cell Sorting) purified using a BD FACSAria II (BD Biosciences) system and BD FACSDiva 8.0.1 software in order to collect EGFP-positive and DAPI negative living cells in 1x PBS containing 10% FBS. The FACS gating strategy is exemplified in Supplementary Fig. 15 . EGFP positive, DAPI negative cells were then centrifuged at 4 °C, 5 min at 300 × g and resuspended in 50 μl of 1x PBS without Ca 2+ and Mg 2+ with 10% FBS. Cells were then loaded in a 10x Chromium instrument (10x Genomics) using the Chromium Single Cell 3’ Library & Reagent kit v2 or single index Chromium Next GEM Single Cell 3’ GEM, Library & Gel Bead kit v3 or v3.1. One scRNA-seq experiment was performed for control and Tbx1 null embryos at E9.5 and two biological replicates were performed for control and Tbx1 null embryos at E10.5. Each sample that was submitted for scRNA-seq was a pool of two or more embryos of the same genotype (Supplementary Table 1 ) Sequencing Sequencing of the DNA libraries was performed using an Illumina HiSeq 4000 system (Genewiz Company, South Plainfield, NY, USA) (scRNA-seq at E9.5 and E10.5) or NovaSeq 6000 system (Novogene, Sacramento, CA, USA) (scRNA-seq at E8.5) with paired-end, 150 bp read length. scRNA-seq data analysis CellRanger (v6.0.1, from 10x Genomics) was used to align scRNA-seq reads to the mouse reference genome (assembly and annotation, mm10-2020-A) to generate gene-by-cell count matrices. All the samples passed quality control measures for Cell Ranger version 6.0.1 (Supplementary Table 1 ). Seurat analysis for filtering and clustering Individual scRNA-seq sample data were analyzed using Seurat V4.0.5 [19] , with parameters as recommended by Seurat software. Integrated scRNA-seq analysis After individual samples were analyzed by Seurat for clustering, the data were integrated by RISC software (v1.6, https://github.com/bioinfoDZ/RISC ) using the Reference Principal Component Integration (RPCI) algorithm for removing batch effects and aligning gene expression values between the control and Tbx1 null samples at E9.5 and E10.5 [40] . 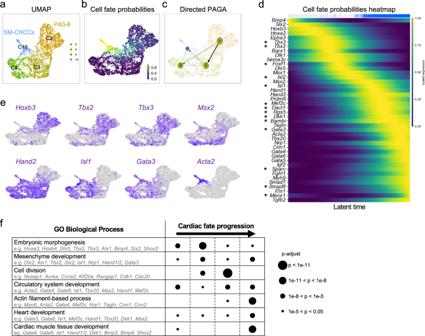Fig. 4: Identification of transition genes and their function at E10.5. aCellRank UMAP plot directed by RNA velocity and cell-cell similarity for clusters C2, C3, C4, and C10 from the feature plot in Fig.3a.bUMAP plot for cell fate probabilities of CNCCs differentiating towards smooth muscle cells.cDirected PAGA plot of NCCs. Pie charts show summarized fate probabilities of individual clusters, with blue representing the proportion of cells in each cluster with high probability to become smooth muscle CNCCs of a cluster, C10.dHeatmap from CellRank showing the expression of selected genes whose expression correlates with transitions of CNCCs fate probabilities, with cells ordered by smooth muscle fate probabilities as latent time (see Supplementary Data5for a full list of genes), Asterisk (*) marks newly identified genes connected to CNCCs.eUMAP plots showing expression of marker genes in CNCCs.fGO enrichment analysis of four groups of genes betweenBmp4andGata6(defined by their pseudotime; Supplementary Data6). Example of genes for each selected GO: biological processes are provided. The size of the dots indicates the adjustedpvalue by Bonferroni and Hochberg correction (Hypergeometric test); adjustedpvalue are indicated in Supplementary Data6. The integrated data were re-clustered by RISC, using parameters adjusted to match the cell type clusters in the Seurat results. 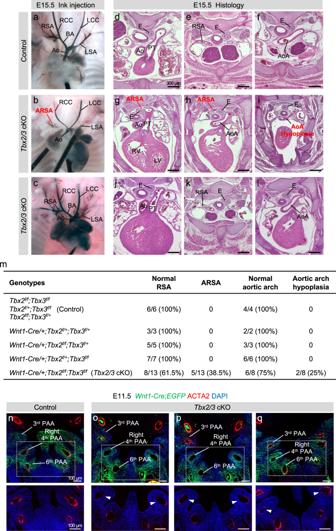Fig. 5:Tbx2andTbx3are required together for aortic arch artery and arterial branching from the aortic arch. a–cIntracardiac ink injection of control (a) (n= 3) andWnt1-Cre;Tbx2f/f;Tbx3f/fconditional null mutant embryos at E15.5 (b,c) (n= 3). Panelbshows a doubleTbx2/Tbx3cKO embryo with an aberrant retro-esophageal right subclavian artery (ARSA).d–lHematotoxin and Eosin staining on traverse sections of control (d,f) (n= 18) andTbx2/Tbx3cKO mutant embryos (g–l) (n= 9) at E15.5. Scale bars: 300 μm. Panelsgandhshow aTbx2/3cKO embryo with ARSA and panelsjandkshow aTbx2/3cKO embryo with a normal right subclavian artery. Panelishows aTbx2/3cKO embryo with aortic arch hypoplasia and panellshows aTbx2/3cKO embryo with a normal aortic arch as compared with control embryos (f).mTable of the cardiovascular defects inTbx2/Tbx3conditional mutants. ARSA was identified in 5/13Tbx2/3cKO embryos: one after intracardiac ink injection, three after H&E histology, and one by anatomic analysis after micro-dissection. Aortic arch hypoplasia was found in 2/8Tbx2/3cKO embryos after H&E histology.n–qImmunofluorescence on coronal sections of controls at E11.5 (n) (n= 8) andTbx2/3cKO embryos (o–q) (n= 8), at the level of the pharyngeal arch arteries for GFP and ACTA2 expression. Nuclei are stained with DAPI. Scale bars: 100 μm. The bottom panels are a high magnification of the dashed regions inn–q. Note the strong reduction of ACTA2 expression, ranging from almost total absence to low-level expression, in the right and left fourth PAAs inTbx2/3conditional mutant embryos compared to control embryos (white arrowheads). RSA right subclavian artery, RCC right common carotid, LCC left common carotid, BA brachiocephalic artery, Ao aorta, AoA aortic arch, LSA left subclavian artery, PT pulmonary trunk, E esophagus, PAA pharyngeal arch artery. Gene expression differences between control and Tbx1 null embryos was determined by RISC software for each of the clusters at an adjusted p value <0.05 and log2 (fold change) >0.25 (using a negative binomial model). 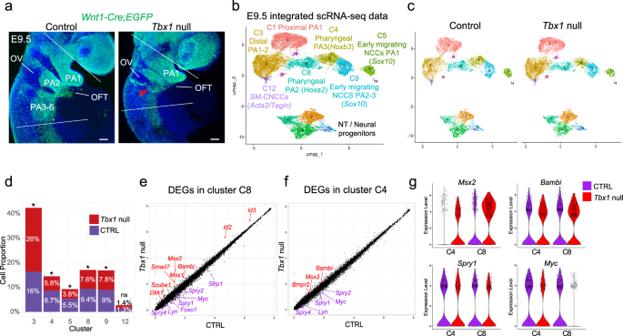Fig. 6: Upregulation of the BMP pathway and downregulation of the MAPK pathway by inactivation ofTbx1at E9.5. aWnt1-Cre;ROSA-EGFPlineage tracing (green) shows mis-localization and a reduced number of NCCs within the pharyngeal region ofTbx1null embryos (red arrow) (n= 10). DAPI is in blue. NCCs from the region between the two dashed lines were used for scRNA-seq.bRISC UMAP plot of integrated scRNA-seq data from NCCs of control andTbx1null embryos.cUMAP plots colored by clusters from control (left) andTbx1null embryos (right).dStack bar graph shows proportions of NCCs in indicated clusters divided by the total number of cells in control orTbx1null embryos. A two-sided proportionz-test was used to evaluate cell proportion differences between control andTbx1null embryos (cluster C3:pvalue = 1.14e-56; C4:pvalue = 9.24e-15; C5:pvalue = 1.46e-8; C8:pvalue = 1.23e-5; C9:pvalue = 4.32e-3; C12:pvalue: 0.66) (*pvalue <0.05; ns not significantly different). Additional information on statistical analysis is provided in the Source Data files.e,fScatter plots show differential gene expression in cluster C8 (e) and in cluster C4 (f) from control andTbx1null embryos. Note the upregulation of genes involved in the BMP pathway (red) and the downregulation of genes in the MAPK pathway (purple).gViolin plots showing differential expression in control (purple) versusTbx1null (red) forMsx2,Bambi,Spry1, andMycin clusters C4 and C8. PA pharyngeal arch, OV otic vesicle, OFT outflow tract. Scale bars: 100 μm. Differentially expressed genes detected in at least 10% of the cells of the clusters of interest were included and those with lower percentages were excluded from the analysis. Cell compositions were computed from the integrated cell clusters and used for the two-proportion Z -test as implemented in the R prop.test() function to evaluate the statistical significance in changes between control and null datasets. At stage E9.5, scRNA-seq was performed with one replicate of control and one replicate of Tbx1 null, with each containing more than one embryo of each genotype. At stage E10.5, we compared the two replicates of control and Tbx1 null scRNA-seq datasets separately and only performed this statistical test for the cell clusters if the directions of the changes were consistent in the two replicates. Cell trajectory analysis CellRank (v1.5.1) [32] was used to infer differentiation trajectory, focusing on determining the probability of cells to adopt the smooth muscle, Acta2 + cell fate. The analysis used RNA velocity from Velocyto (v0.17.17) [83] and scVelo (v0.2.4) [83] , as well as cell-cell similarity, to infer trajectories and cell differentiation potential. The analysis was performed for all cells in either the E9.5 control sample or the two E10.5 control samples and then for the cells in the selected clusters that were predicted to have connections to the smooth muscle Acta2 + cluster. 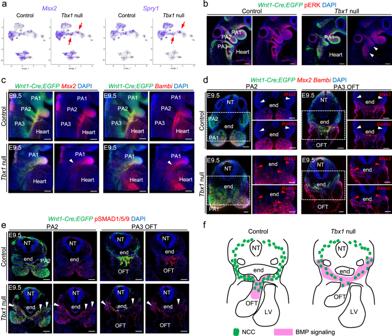Fig. 7: BMP pathway is downregulated and the MAPK pathway is upregulated in pharyngeal NCCs ofTbx1null embryos at E9.5. aUMAP plots show the expression level (purple) ofMsx2andSpry1in NCCs split by control andTbx1null embryos.bWholemount immunostaining throughWnt1-Cre;ROSA-EGFPcontrol (n= 7) andTbx1null embryos (n= 5) for GFP (green) and phospho-ERK (pERK) (red). Digitally generated sections are shown inb. DAPI is in blue. Arrowheads show reduced expression of pERK in NCCs in the pharyngeal region ofTbx1null embryo.cMsx2,Bambi, andEgfpwholemount RNAscope in situ hybridization with DAPI of control andTbx1null embryos. (Msx2in control:n= 7,Msx2inTbx1null embryos:n= 3,Bambiin control andTbx1null embryo:n= 3) The arrowheads indicate ectopic expression ofMsx2andBambiinTbx1null embryos.dEgfp,Msx2, andBambiRNAscope assay on transverse sections of control andTbx1null embryos (n= 3) showing ectopic and dorsal expression ofMsx2andBambiin migrating NCCs (red arrowheads).Msx2andBambiexpression is absent in the proximal part of the PA2 and PA3 of control embryos (white arrowheads).eFluorescent immunostaining for GFP and P-SMAD1/5/9 on transverse sections of control (n= 5) andTbx1null (n= 4) embryos shows increase in P-SMAD1/5/9 in NCCs of PA2-3 (arrowheads).fSchematic representation of control (left) andTbx1null (right) sections at E9.5 showing reduced CNCCs contributing to the shortened OFT and ectopic posterior BMP signaling. PA pharyngeal arch, OFT outflow tract, NT neural tube, end endoderm, LV left ventricle. Scale bars: 100 μm. Cell-cell communication analysis CellChat (v1.1.3) [44] was used to identify the ligand–receptor interactions between Mesp1 Cre mesoderm lineage and NCC lineages and then compare the change between control and Tbx1 null mutant data at p < 0.05. Data included ligands in the Mesp1 Cre lineage and receptors in the CNCC lineage. Mesp1 Cre control and Tbx1 conditional null datasets were integrated with RISC software for clustering and dimension reduction using cell type annotation as previously described in ref. 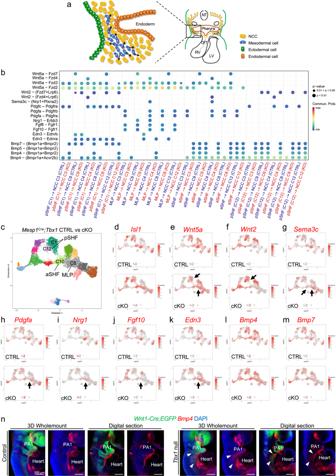Fig. 8: Cell-cell communication from the mesoderm to NCCs is altered in the absence ofTbx1at E9.5. aSchematic representation of a transverse section showing signaling (arrows) from pharyngeal mesoderm cells (blue) to NCCs (yellow) in the caudal pharyngeal apparatus.bBubble plot shows representative cell-cell signaling fromMesp1Crederived mesodermal cells to NCCs that were significantly altered (Wilcox rank two-sided test without multiple test correction,pvalue indicated by the size of dot and color; right) inTbx1mutant embryos. Each dot represents a ligand–receptor pair interaction (Y-axis) between a specific cluster in the mesoderm cells and NCCs (X-axis). Clusters include anterior and posterior second heart fields (aSHF, pSHF) and the multilineage progenitors (MLP).cUMAP from integration of two replicates ofMesp1Cre;ROSA-EGFP(CTRL) andMesp1Cre;Tbx1f/f;EGFP(Tbx1cKO) datasets.dUMAP plots showingIsl1expression in control andTbx1cKO cells.e–mUMAP plots showing the expression of ligand genes includingWnt5a(e),Wnt2(f),Sema3c(g),Pdgfa(h),Nrg1(i),Fgf10(j),Edn3(k),Bmp4(l), andBmp7(m) incontrolandTbx1cKO embryos. Arrows indicate cell clusters with gene expression changes inTbx1cKO embryos.nWholemount RNAscope in situ hybridization ofWnt1-Cre;ROSA-EGFPcontrol (lefts panels) andTbx1null (right panels) embryos at E9.5 with probes forEgfpandBmp4. Representative digital sections are shown on the right of 3D reconstruction pictures. Arrowheads show expression ofBmp4in cells adjacent to the pharyngeal NCCs inTbx1null embryos. PA pharyngeal arch. Scale bars: 200 μm. [46] . 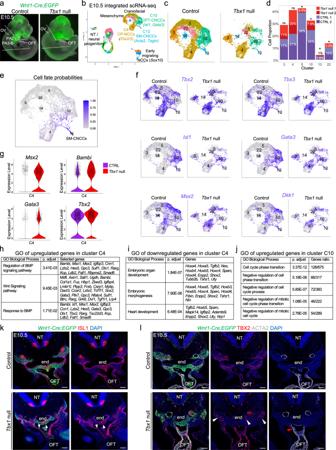Fig. 9: Failure of CNCC cell fate progression by loss ofTbx1at E10.5. aThe NCCs between the dotted lines and heart in control andTbx1null embryos were used for scRNA-seq.bRISC UMAP plot of integrated scRNA-seq data from NCCs of two replicates of control andTbx1null embryos.cUMAP plots of pharyngeal and heart clusters from control (left) andTbx1null (right) embryos.dStack bar graph shows proportions of NCCs in selected clusters divided by the total cell number in control orTbx1null replicates. A two-sided proportionz-test was used to evaluate cell proportion differences between control andTbx1null embryos for the two replicates separately if the twoTbx1null show consistent increase or decrease compared to control. (*pvalue <0.05; ns not significantly different, see Source Data file forpvalue details).eUMAP plot colored by cell fate probabilities.fUMAP plots showing expression level ofTbx2,Tbx3,Isl1, Gata3,Msx2, andDkk1in NCCs from control orTbx1null embryos in pharyngeal NCC clusters.Msx2,Gata3, andDkk1show increased expression in cluster C4.gViolin plots showing differential expression level ofMsx2,Bambi,Gata3, andTbx2in cluster C4 in control (purple) andTbx1null (red) embryos.h–jGO analysis for upregulated genes in C4 (h), downregulated genes in C4 (i), and upregulated genes in C10 (j). Hypergeometric test was used, adjustedpvalue by Bonferroni–Hochberg correction.kFluorescent immunostaining for GFP (green) and ISL1 (red) with DAPI (blue) on transverse sections of control (n= 4) andTbx1null (n= 3) embryos. There is reduced ISL1-positive NCCs (arrowheads).lFluorescent immunostaining for GFP (green), TBX2 (red), and ACTA2 (gray) on transverse sections of control (n= 4) andTbx1null (n= 3) embryos, DAPI is in blue. Expression of TBX2 in NCCs is lateral to the pharyngeal endoderm (end; white arrowheads). There are fewer CNCCs expressing ACTA2 within the OFT ofTbx1null embryos (red arrowhead). NT neural tube, end endoderm, OFT outflow tract. Scale bars: 100 μm. 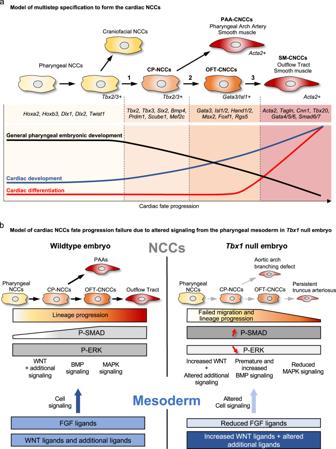Fig. 10: Model of a multistep specification to form CNCCs and the signaling pathways disrupted by inactivation ofTbx1. aColors indicate cell fate progression of pharyngeal NCCs (light yellow) towards vascular smooth muscle cells (red). Step 1 shows the transition between pharyngeal NCCs expressingTbx2/3to cells expressing markers of CNCCs (CP-CNCCs). Step 2 shows the transition in which some cells directly differentiate to smooth muscle of PAA-CNCCs, while the majority migrate and enter the OFT as OFT-CNCCs and expressGata3/Isl1and Step 3 shows the transition to SM-CNCCs expressingActa2. The graph shows the relative change of biological gene ontology terms during the three transitions of CNCCs to smooth muscle cells.bModel of non-autonomous signaling between the mesoderm (bottom, blue) and NCCs (top, gray) highlighting FGF, WNT, and additional signaling from the mesoderm to NCCs in normal embryos (left) and how signaling is disrupted in the absence ofTbx1(light blue arrows/inhibitory arrows; right). Alteration of signaling in the mesoderm in the absence ofTbx1results in abnormal premature activation of the BMP pathway during NCC deployment and migration (light blue inhibitory arrow; red, up arrow), a decrease of MAPK signaling in NCCs (light blue arrow; red down arrow), and alteration of other signaling pathways including upregulation of WNT signaling in developing NCCs. This leads to failure of cardiac fate progression with a reduced number of CP-CNCCs, reduced number of CNCCs, and reduced number of SM-CNCCs (gray arrows) with aortic arch/branching defects and failed OFT septation (persistent truncus arteriosus). Reporting summary Further information on research design is available in the Nature Portfolio Reporting Summary linked to this article.